O-Linked-N-acetylglucosamine on extracellular protein domains mediates epithelial cell–matrix interactions The O-linked- N -acetylglucosamine (O-GlcNAc) modification of cytoplasmic and nuclear proteins regulates basic cellular functions and is involved in the aetiology of diabetes and neurodegeneration. This intracellular O-GlcNAcylation is catalyzed by a single O-GlcNAc transferase, OGT. Here we report a novel OGT, EOGT, responsible for extracellular O-GlcNAcylation. Although both OGT and EOGT are regulated by hexosamine flux, EOGT localizes to the lumen of the endoplasmic reticulum and transfers GlcNAc to epidermal growth factor-like domains in an OGT-independent manner. Loss of Eogt gives phenotypes similar to those caused by defects in the apical extracellular matrix. Dumpy (Dp), a membrane-anchored extracellular protein, is O-GlcNAcylated, and EOGT is required for Dp-dependent epithelial cell–matrix interactions. Thus, O-GlcNAcylation of secreted and membrane glycoproteins is a novel mediator of cell–cell or cell–matrix interactions at the cell surface. O-Linked- N -acetylglucosamine (O-GlcNAc) modification is a unique post-translational modification that cooperates with phosphorylation to regulate a variety of cellular processes, including intracellular signalling, cytokinesis, transcription and protein stability, and serves to modulate nutrient sensing [1] , [2] , [3] . O-GlcNAcylation is also involved in epigenetic control of cell differentiation and is implicated in the aetiology of several human diseases, including type 2 diabetes and neurodegeneration [4] , [5] , [6] . Although many reports have described biological roles of O-GlcNAcylation, they were limited to the intracellular protein functions [7] , as the modification had been believed to be restricted to the cytoplasm and nucleus [7] . However, a few reports have identified O-GlcNAc in the extracellular environment [8] , [9] . Nevertheless, this could be attributed to a non-canonical secretion pathway for proteins that bypass the endoplasmic reticulum (ER) and Golgi compartments [7] . To date, a sole O-GlcNAc transferase, OGT [10] , has been shown to catalyze intracellular O-GlcNAcylation [11] , [12] . Here we show that O-GlcNAc is expressed in the apical extracellular matrix (aECM) and that it is required for epithelial cell adhesion/interaction with the ECM in Drosophila . This cell–matrix interaction is mediated by a novel ER-resident O-GlcNAc transferase, EOGT. This enzyme is responsible for O-GlcNAcylation of proteins in the secretory pathway independently of OGT activity. Dumpy (Dp), a membrane-anchored extracellular protein, is O-GlcNAcylated, and EOGT mediates cell–matrix interactions in a Dp-dependent manner. These findings reveal new biological roles for O-GlcNAcylation in secreted and membrane glycoproteins and the extracellular environment. EOGT is required for extracellular O-GlcNAcylation O-GlcNAc transferase activity responsible for modifying the epidermal growth factor (EGF) repeats in the extracellular domain of Notch was previously detected in the membrane fraction of Drosophila S2 cells [9] . We performed an RNA interference (RNAi)-based search for genes that specifically affect O-GlcNAcylation by following changes in glycosylation by matrix-assisted laser desorption/ionization–time of flight-mass spectrometry. As other Notch O-glycosyltransferases are ER-resident proteins [13] , [14] , [15] , we initiated screening by targeting putative glycosyltransferases possessing an ER retention signal, which are listed in the CAZy database ( http://www.cazy.org ). S2 cells were treated with double-stranded RNA (dsRNA) corresponding to the selected gene and simultaneously transfected to express Notch EGF domain 20 (EGF20). We identified one candidate gene, EOGT (EGF-domain O-GlcNAc transferase; Supplementary Fig. S1 ), whose downregulation decreased the signals corresponding to O-GlcNAcylated EGF20 peptides ( Fig. 1a,b and Supplementary Fig. S2 ). EOGT is conserved from Drosophila to mammals ( Fig. 1c ), but shows no apparent homology to previously isolated GlcNAc-transferases, such as OGT or GlcNAcT enzymes. Co-expression of FLAG (DYKDDDDK)-tagged Notch EGF repeats (N-EGF:FLAG) with EOGT or other selected genes revealed that EOGT specifically elevates the O-GlcNAc level on EGF domains ( Fig. 1d ). Furthermore, O-GlcNAcylation of endogenous Notch was nearly eliminated by Eogt RNAi ( Fig. 1e ). Thus, EOGT retains an activity required for extracellular O-GlcNAcylation. 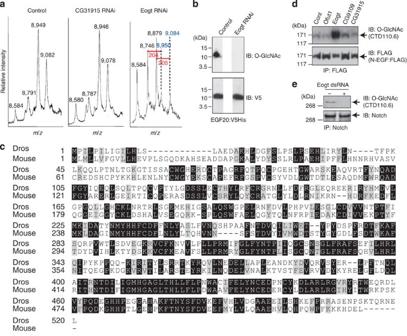Figure 1: Identification of an EGF domain-specific O-GlcNAc transferase, EOGT. (a) Matrix-assisted laser desorption/ionization–time of flight mass spectrum of Notch EGF20 prepared from culture media of wild-type or dsRNA-treated S2 cells. S2 cells untreated or treated with dsRNA corresponding to CG31915 orEogtwere transiently transfected with a construct encoding EGF20:V5His. After affinity-purification using Ni-magnetic beads, proteins were analyzed by MALDI-TOF-MS using the 4700 Proteomic Analyzer in the linear positive mode as described previously9. The mass/charge (m/z) values are shown in bold numbers. Peak-to-peak mass increment corresponding to O-GlcNAc modification is indicated by double-headed red arrows. The theoretical average mass for a singly charged and unglycosylated EGF20 peptide with three disulphide bonds is 8,438. (b) Notch EGF20 fragments purified from culture media of S2 cells treated without or withEogtdsRNA were subjected to immunoblotting (IB) with CTD110.6 (O-GlcNAc) and V5 antibodies. (c) Alignment of amino-acid sequences ofDrosophilaand mouse EOGT. Black-shaded residues indicate identity; grey-shaded residues indicate similarity. (d) Immunoblot analysis for O-GlcNAcylation of N-EGF:FLAG isolated from the medium of S2 cells. Cells were co-transfected with the indicated constructs. IP, immunoprecipitation. (e) Effect ofEogtRNAi on O-GlcNAcylation of endogenous Notch. Proteins immunoprecipitated from Kc cell lysates with anti-Notch antibody were detected by anti-O-GlcNAc antibody. Figure 1: Identification of an EGF domain-specific O-GlcNAc transferase, EOGT. ( a ) Matrix-assisted laser desorption/ionization–time of flight mass spectrum of Notch EGF20 prepared from culture media of wild-type or dsRNA-treated S2 cells. S2 cells untreated or treated with dsRNA corresponding to CG31915 or Eogt were transiently transfected with a construct encoding EGF20:V5His. After affinity-purification using Ni-magnetic beads, proteins were analyzed by MALDI-TOF-MS using the 4700 Proteomic Analyzer in the linear positive mode as described previously [9] . The mass/charge ( m / z ) values are shown in bold numbers. Peak-to-peak mass increment corresponding to O-GlcNAc modification is indicated by double-headed red arrows. The theoretical average mass for a singly charged and unglycosylated EGF20 peptide with three disulphide bonds is 8,438. ( b ) Notch EGF20 fragments purified from culture media of S2 cells treated without or with Eogt dsRNA were subjected to immunoblotting (IB) with CTD110.6 (O-GlcNAc) and V5 antibodies. ( c ) Alignment of amino-acid sequences of Drosophila and mouse EOGT. Black-shaded residues indicate identity; grey-shaded residues indicate similarity. ( d ) Immunoblot analysis for O-GlcNAcylation of N-EGF:FLAG isolated from the medium of S2 cells. Cells were co-transfected with the indicated constructs. IP, immunoprecipitation. ( e ) Effect of Eogt RNAi on O-GlcNAcylation of endogenous Notch. Proteins immunoprecipitated from Kc cell lysates with anti-Notch antibody were detected by anti-O-GlcNAc antibody. Full size image EOGT encodes an EGF domain O-GlcNAc transferase To investigate whether EOGT itself has O-GlcNAc transferase activity, we isolated V5-hexahistidine-tagged EOGT (EOGT:V5His) from the membrane fraction of cultured S2 cells. The membrane fraction proteins or purified EOGT:V5His was incubated with yeast-expressed unglycosylated EGF20 and uridine diphosphate (UDP)-[ 3 H]GlcNAc in buffer. Transfer of [ 3 H]GlcNAc to EGF20 was detected only in the presence of EOGT:V5His ( Fig. 2a,b ). Divalent cations, especially Mn 2+ , stimulated EOGT activity, although they were not absolutely required ( Fig. 2c,d ). Lack of a requirement for Mn 2+ has been reported in a subset of glycosyltransferases, including GlcNAcT-V [16] and plant β2-xylosyltransferase [17] . EOGT shows partial homology to the β2-xylosyltransferase (19.4% identity to Arabidopsis thaliana β2-xylosyltransferase), suggesting that EOGT and the plant enzyme share common structural features. Analysis of donor substrate specificity revealed that EOGT uses UDP-GlcNAc, but not UDP-GalNAc, a sugar donor for mucin-type O-glycosylation ( Fig. 2e ). As acceptor substrates, folded EGF domains, but not structurally altered variants of EGF20, served as good substrates. EGF20 ΔGlcΔFuc (lacking O-glucosylation and O-fucosylation sites) was also GlcNAcylated by EOGT, albeit less efficiently than wild-type EGF20, whereas EGF20 T34A (a mutation of Thr34, the O-glycosylation site in EGF20, to Ala) was not detectably O-GlcNAcylated ( Fig. 2e and Supplementary Fig. S3 ). Thus, EOGT is an EGF domain O-GlcNAc transferase that specifically modifies Thr34 of EGF20. 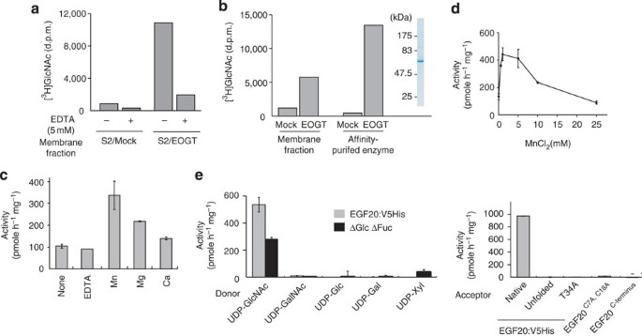Figure 2: Detection and characterization of O-GlcNAc transferase activity of EOGT. (a,b)In vitroglycosylation assays. O-GlcNAc transferase activity was measured using membrane fraction proteins or affinity-purified proteins, recombinant EGF20 prepared from yeast and UDP-[3H]GlcNAc. (a) S2 cells were transfected with or without a construct expressing EOGT:V5His, and membrane fraction proteins were used for enzyme source. Reactions were performed in either the presence or absence of 5 mM EDTA. (b) S2 cells were transfected with or without a construct expressing EOGT:V5His, and membrane fraction proteins were used for enzyme source. Where indicated, membrane fraction proteins were further purified with Ni-magnetic beads. CBB staining of the purified enzyme is also shown (right). (c) Metal requirements of EOGT:V5His. (d) Effect of increasing concentration of MnCl2on O-GlcNAc transferase activity. (e) Donor (left) and acceptor (right) specificity of EOGT:V5His. (c–e) Vertical bars represent a range of values obtained from duplicate samples. At least three experiments were performed, which each gave the similar results. Figure 2: Detection and characterization of O-GlcNAc transferase activity of EOGT. ( a , b ) In vitro glycosylation assays. O-GlcNAc transferase activity was measured using membrane fraction proteins or affinity-purified proteins, recombinant EGF20 prepared from yeast and UDP-[ 3 H]GlcNAc. ( a ) S2 cells were transfected with or without a construct expressing EOGT:V5His, and membrane fraction proteins were used for enzyme source. Reactions were performed in either the presence or absence of 5 mM EDTA. ( b ) S2 cells were transfected with or without a construct expressing EOGT:V5His, and membrane fraction proteins were used for enzyme source. Where indicated, membrane fraction proteins were further purified with Ni-magnetic beads. CBB staining of the purified enzyme is also shown (right). ( c ) Metal requirements of EOGT:V5His. ( d ) Effect of increasing concentration of MnCl 2 on O-GlcNAc transferase activity. ( e ) Donor (left) and acceptor (right) specificity of EOGT:V5His. ( c – e ) Vertical bars represent a range of values obtained from duplicate samples. At least three experiments were performed, which each gave the similar results. Full size image EOGT is involved in OGT-independent O-GlcNAcylation The hexosamine pathway of glucose metabolism leads to UDP-GlcNAc synthesis [1] . As UDP-GlcNAc serves as a sugar donor for both OGT and EOGT, we investigated whether extracellular O-GlcNAcylation is linked to OGT-dependent glycosylation. Glutamine:fructose-6-phosphate aminotransferase is a rate-limiting enzyme for glucose entry into the hexosamine pathway. Exogenous GlcNAc can bypass this step, directly entering the hexosamine pathway and being converted to UDP-GlcNAc. Supplementing the medium with GlcNAc markedly increased O-GlcNAc levels on endogenous Notch and bulk intracellular proteins, suggesting that both intracellular and extracellular O-GlcNAcylations are controlled by a common hexosamine pathway ( Fig. 3a ). However, Eogt RNAi nearly eliminated O-GlcNAcylation of secreted N-EGF:FLAG, whereas O-GlcNAcylation of intracellular proteins was unaffected. Conversely, Ogt RNAi or inhibition of O-GlcNAcase by PUGNAc affected intracellular, but not extracellular, O-GlcNAc levels ( Fig. 3b ). Thus, OGT and EOGT act selectively and independently to control intracellular and extracellular O-GlcNAcylation, respectively. 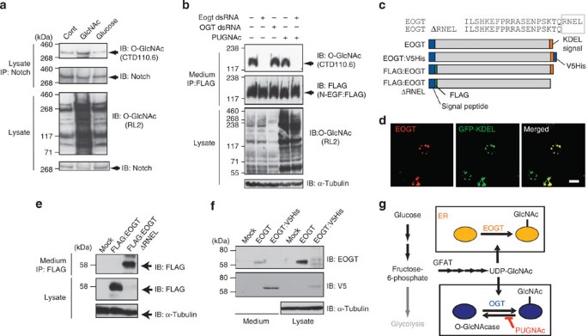Figure 3: EOGT is involved in OGT-independent O-GlcNAcylation. (a) Immunoblot analysis for O-GlcNAcylation of whole-cell lysates (RL-2) or anti-Notch immunoprecipitants (CTD110.6) of Kc cells; the cells were cultured with the indicated supplements. (b) Immunoblot analysis for O-GlcNAcylation of N-EGF:FLAG isolated from the medium and whole-cell lysates of S2 cells; the cells were treated with indicated dsRNAs or PUGNAc. (c) Schematics of EOGT constructs and C-terminal sequences, with proposed KDEL signal boxed. (d) Confocal images of S2 cells transfected with GFP:KDEL and EOGT. Scale bar, 20 μm. (e) S2 cells were transfected with control vector (Mock), constructs expressing FLAG:EOGT or FLAG:EOGTΔRNEL. Ability of the cells to retain each construct was analyzed by immunoblotting of cell lysates and FLAG-tag purified secreted proteins. Immunoblot with anti-FLAG antibody revealed the mislocalization of FLAG:EOGTΔRNEL. (f) S2 cells were transfected with control vector (Mock), or constructs expressing EOGT or EOGT:V5His. Ability of the cells to retain each construct was analyzed by immunoblotting (IB) of cell lysates and secreted proteins using EOGT and V5 antibodies. Note that addition of V5His tag to EOGT precludes detection by EOGT antibody. (g) Schematic of the EOGT-dependent O-GlcNAcylation pathway. GFAT, glutamine:fructose-6-phosphate aminotransferase;IP, immunoprecipitation. Figure 3: EOGT is involved in OGT-independent O-GlcNAcylation. ( a ) Immunoblot analysis for O-GlcNAcylation of whole-cell lysates (RL-2) or anti-Notch immunoprecipitants (CTD110.6) of Kc cells; the cells were cultured with the indicated supplements. ( b ) Immunoblot analysis for O-GlcNAcylation of N-EGF:FLAG isolated from the medium and whole-cell lysates of S2 cells; the cells were treated with indicated dsRNAs or PUGNAc. ( c ) Schematics of EOGT constructs and C-terminal sequences, with proposed KDEL signal boxed. ( d ) Confocal images of S2 cells transfected with GFP:KDEL and EOGT. Scale bar, 20 μm. ( e ) S2 cells were transfected with control vector (Mock), constructs expressing FLAG:EOGT or FLAG:EOGT ΔRNEL . Ability of the cells to retain each construct was analyzed by immunoblotting of cell lysates and FLAG-tag purified secreted proteins. Immunoblot with anti-FLAG antibody revealed the mislocalization of FLAG:EOGT ΔRNEL . ( f ) S2 cells were transfected with control vector (Mock), or constructs expressing EOGT or EOGT:V5His. Ability of the cells to retain each construct was analyzed by immunoblotting (IB) of cell lysates and secreted proteins using EOGT and V5 antibodies. Note that addition of V5His tag to EOGT precludes detection by EOGT antibody. ( g ) Schematic of the EOGT-dependent O-GlcNAcylation pathway. GFAT, glutamine:fructose-6-phosphate aminotransferase;IP, immunoprecipitation. Full size image EOGT localizes to the lumen of the ER We next examined whether the distinct roles of OGT and EOGT are derived from their different subcellular localization. As expected from its signal peptide and carboxyl-terminal KDEL-like sequence RNEL ( Fig. 3c ), EOGT localized in organelles that co-stained with the ER marker GFP-KDEL ( Fig. 3d ). Expression of a construct lacking the RNEL sequence (EOGT ΔRNEL ) or C-terminally tagged with V5His (EOGT:V5His) resulted in a marked shift in localization from cell lysate to culture medium ( Fig. 3e,f ), suggesting that the KDEL-like sequence serves as an ER retrieval signal. Thus, EOGT is a soluble ER protein that catalyzes OGT-independent O-GlcNAcylation of secreted and membrane glycoproteins ( Fig. 3g ). Mutation of Eogt causes defects in the aECM To explore the biological events associated with extracellular O-GlcNAcylation, we generated Drosophila mutants of Eogt ( Fig. 4a and Supplementary Fig. S4 ). In situ hybridization study revealed that the highest expression of Eogt , likely the maternal contribution, was observed in preblastoderm-stage embryos ( Fig. 4b ). At later stages of embryogenesis, the expression is ubiquitous but the expression level decreases as the stage proceeds ( Fig. 4c–e ). Strikingly, although mutants lacking both maternal and zygotic (M/Z) expression of Eogt failed to hatch, but no apparent defect was observed in Notch-dependent neurogenesis ( Fig. 4f ), and the pattern of somatic musculature was unchanged ( Fig. 4g ). However, after muscle contraction during late stage 17, all segments were compacted and the muscle bands were correspondingly shorter ( Fig. 4h,i ), suggesting that Eogt is essential during embryogenesis, but in a Notch-independent manner. 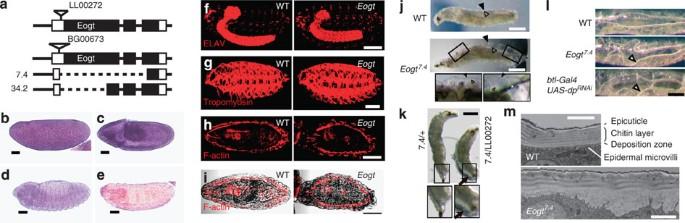Figure 4: Generation and characterization ofDrosophila Eogtmutants. (a) Schematic of theEogtlocus. Exons (bars) and the open reading frame (black bars) are depicted. BothEogt7.4andEogt34.2lack sequences corresponding to the translational start codon (ATG197), signal peptide and a portion of the catalytic domain (∼Phe395inEogt7.4and∼Thr222inEogt34.2) that are highly conserved fromDrosophilaand mammals. Thus, these two lines are expected to be null alleles. (b–e)In situhybridization analysis ofEogtexpression during embryogenesis. (b) The highest expression ofEogt, likely the maternal contribution, was observed in preblastoderm-stage embryos. (c), Stage 11; (d), stage 13; (e), stage 16 embryos. Scale bars, 50 μm. (f) Wild-type (WT) andEogt7.4embryos lacking maternal and zygotic expression (EogtM/Zembryos) were stained for the neuronal marker ELAV. (g) Stage 16 WT andEogtM/Zembryos stained for tropomyosin. (h) Stage 17 WT andEogtM/Zembryos were stained with phalloidin. (i) An overlay of the differential interference contrast (DIC) and fluorescence image shown inh. (f–i) Scale bars, 100 μm. (j) Live images of WT andEogt7.4homozygous second-instar larvae. Enlargement of the boxed area is shown below. InEogt7.4larvae, cuticles were partially detached from the epidermis (arrowheads), although the larval body was not compacted and the body size was comparable with that of the WT larvae. The trachea remains attached to posterior spiracles (asterisk). Scale bars, 400 μm. (k) Cuticle detachment ofEogt7.4/LL00272third-instar larvae. Enlargement of the boxed area is shown below. Scale bar, 500 μm. (l) Tracheal morphology of WT,Eogt7.4mutant andbtl-Gal4 UAS-dpRNAisecond-instar larvae. Dorsal view of larvae with similar body length and diameter is shown. Scale bar, 200 μm. In theEogt7.4mutant andbtl-Gal4 UAS-dpRNAilarvae, the tracheae are distorted relative to the WT larvae (arrowheads). (m) Ultrastructural images of WT andEogt7.4homozygous second-instar larvae. Scale bar, 2 μm. Figure 4: Generation and characterization of Drosophila Eogt mutants. ( a ) Schematic of the Eogt locus. Exons (bars) and the open reading frame (black bars) are depicted. Both Eogt 7.4 and Eogt 34.2 lack sequences corresponding to the translational start codon (ATG 197 ), signal peptide and a portion of the catalytic domain ( ∼ Phe 395 in Eogt 7.4 and ∼ Thr 222 in Eogt 34.2 ) that are highly conserved from Drosophila and mammals. Thus, these two lines are expected to be null alleles. ( b – e ) In situ hybridization analysis of Eogt expression during embryogenesis. ( b ) The highest expression of Eogt , likely the maternal contribution, was observed in preblastoderm-stage embryos. ( c ), Stage 11; ( d ), stage 13; ( e ), stage 16 embryos. Scale bars, 50 μm. ( f ) Wild-type (WT) and Eogt 7.4 embryos lacking maternal and zygotic expression ( Eogt M/Z embryos) were stained for the neuronal marker ELAV. ( g ) Stage 16 WT and Eogt M/Z embryos stained for tropomyosin. ( h ) Stage 17 WT and Eogt M/Z embryos were stained with phalloidin. ( i ) An overlay of the differential interference contrast (DIC) and fluorescence image shown in h . ( f–i ) Scale bars, 100 μm. ( j ) Live images of WT and Eogt 7.4 homozygous second-instar larvae. Enlargement of the boxed area is shown below. In Eogt 7.4 larvae, cuticles were partially detached from the epidermis (arrowheads), although the larval body was not compacted and the body size was comparable with that of the WT larvae. The trachea remains attached to posterior spiracles ( asterisk ). Scale bars, 400 μm. ( k ) Cuticle detachment of Eogt 7.4/LL00272 third-instar larvae. Enlargement of the boxed area is shown below. Scale bar, 500 μm. ( l ) Tracheal morphology of WT, Eogt 7.4 mutant and btl-Gal4 UAS-dp RNAi second-instar larvae. Dorsal view of larvae with similar body length and diameter is shown. Scale bar, 200 μm. In the Eogt 7.4 mutant and btl-Gal4 UAS-dp RNAi larvae, the tracheae are distorted relative to the WT larvae (arrowheads). ( m ) Ultrastructural images of WT and Eogt 7.4 homozygous second-instar larvae. Scale bar, 2 μm. Full size image The morphological defects in Eogt M/Z embryos are similar to mutants for Piopio (Pio), a zona pellucida (ZP) protein required for the integrity of the aECM (known as cuticle) [18] . Embryos lacking ZP proteins such as Papillote, Dp and Pio show a defect in the formation of the innermost layer of the aECM and its attachment to the epidermis [19] . Eogt 7.4 homozygotes and Eogt 7.4/LL00272 transheterozygotes died mostly during second-instar or second/third-instar interface, but some survived until early third-instar. Those Eogt mutant larvae displayed cuticle defect ( Fig. 4j,k ) and irregular tracheal morphology, which appears to correspond to the defects observed in dp mutants ( Fig. 4l ) [19] , [20] . Ultrastructural analysis of larval epidermis revealed disruption of the deposition zone of the endocuticle, leading to separation of the epidermis from the chitin layers ( Fig. 4m ). These results suggest that Eogt contributes to the aECM or its link to the epidermis. The integrity of aECM is also required for the flat morphology of adult wings, and deficiency in the aforementioned ZP proteins or Eogt results in wing blistering ( Supplementary Fig. S5 ) [19] , [21] . Although deficiencies in integrin-dependent epithelial cell contact with basal ECM also causes wing blistering, βPS integrin activity and localization were unaffected by EOGT removal ( Supplementary Fig. S6a,b ). Eogt does not interact genetically with mys (βPS integrin; Supplementary Fig. S6c ), and muscle detachment, a characteristic loss-of-function phenotype for integrin, was not observed in Eogt embryos ( Fig. 4g–i ). These results suggest that EOGT mediates adhesion of the wing epithelium in an integrin function-independent manner. EOGT O-GlcNAcylates Dp Among the aforementioned ZP proteins, only Dp, a giant 2.5 MDa membrane-anchored extracellular protein, contains EGF-like domains and a very large number of them (308 EGF-like repeats; Fig. 5a,b ) [22] . Immunoblotting of cuticle extracts revealed that O-GlcNAcylation occurs almost exclusively on a single high-molecular-weight protein, which was identified as Dp by immunoprecipitation analysis ( Fig. 5c,d ). In contrast, glycosylation of the other O-GlcNAcylated proteins detected in total larval lysates was not impaired in Eogt mutants ( Fig. 5e and Supplementary Fig. S2 ). This supports our proposal that EOGT does not affect OGT-dependent intracellular O-GlcNAcylation. Partial fragments of EGF–DPY–EGF repeats of Dp expressed in S2 cells demonstrated that EGF94–103 and EGF108–117, but not EGF84–93, are O-GlcNAcylated. Moreover, depletion of EOGT by RNAi yielded a marked decrease in the O-GlcNAc level ( Fig. 5f,g and Supplementary Fig. S2 ). The remaining O-GlcNAc signal in EGF94–103 is because of the residual enzyme activity in EOGT-depleted cells as no EOGT homologues are present in Drosophila . Alignment of these sequences with Notch EGF20 suggested that Thr/Ser residues located at the fifth position after the fifth conserved Cys residue are O-GlcNAc modification sites ( Fig. 5b ). Consistently, Ala substitutions of the putative glycosylation sites of EGF94-103 and EGF108-117 (ΔGlcNAc) abrogated O-GlcNAcylation ( Fig. 5f and Supplementary Fig. S2 ). Although the precise O-GlcNAcylation sites on Dp have not yet been mapped experimentally, these data clearly showed that C 5 XXXX T/S G is the modification site for O-GlcNAcylation of EGF domains, and that up to 86 EGF domains could be O-GlcNAcylated ( Supplementary Fig. S7 ). Interestingly, these modification sites are mostly located within the second EGF-like domain of the EGF–DPY–EGF repeats. 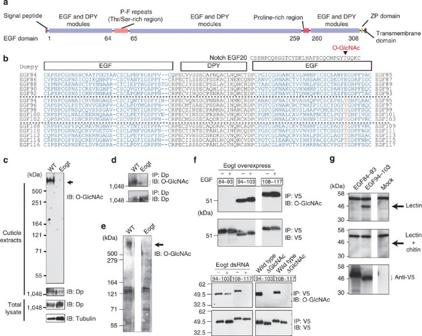Figure 5: EOGT O-GlcNAcylates Dumpy. (a) Schematic representation of the structure of Dp. (b) Partial alignment of EGF–DPY–EGF repeats of Dp. O-GlcNAcylation sites are shown in red. (c) Immunoblot analysis of total lysates and cuticle extracts prepared from wild-type (WT) andEogt7.4second-instar larvae. (d) Immunoblot analysis of anti-Dp immunoprecipitants isolated from cuticle extracts of WT andEogt7.4second-instar larvae. (e) Immunoblot analysis of total lysates prepared from WT andEogt7.4second-instar larvae. O-GlcNAcylation of a high-molecular-weight protein is specifically affected inEogtmutants (arrow). (f) Immunoblot analysis of Dp fragments and the mutants lacking O-GlcNAcylation sites (ΔGlcNAc) isolated from the medium of S2 cells. Where indicated,Eogtis exogenously expressed or silenced by dsRNA treatment. (g) O-GlcNAcylated Dp fragments bind to a plant chitin-binding lectin, wheat germ agglutinin (WGA). Isolated Dp fragments were subjected to lectin blotting with/without chitin hydrolysates. O-GlcNAc on Dp has the ability to associate with WGA, and binding is inhibited by chitin. IB, immunoblotting; IP, immunoprecipitation. Figure 5: EOGT O-GlcNAcylates Dumpy. ( a ) Schematic representation of the structure of Dp. ( b ) Partial alignment of EGF–DPY–EGF repeats of Dp. O-GlcNAcylation sites are shown in red. ( c ) Immunoblot analysis of total lysates and cuticle extracts prepared from wild-type (WT) and Eogt 7.4 second-instar larvae. ( d ) Immunoblot analysis of anti-Dp immunoprecipitants isolated from cuticle extracts of WT and Eogt 7.4 second-instar larvae. ( e ) Immunoblot analysis of total lysates prepared from WT and Eogt 7.4 second-instar larvae. O-GlcNAcylation of a high-molecular-weight protein is specifically affected in Eogt mutants (arrow). ( f ) Immunoblot analysis of Dp fragments and the mutants lacking O-GlcNAcylation sites (ΔGlcNAc) isolated from the medium of S2 cells. Where indicated, Eogt is exogenously expressed or silenced by dsRNA treatment. ( g ) O-GlcNAcylated Dp fragments bind to a plant chitin-binding lectin, wheat germ agglutinin (WGA). Isolated Dp fragments were subjected to lectin blotting with/without chitin hydrolysates. O-GlcNAc on Dp has the ability to associate with WGA, and binding is inhibited by chitin. IB, immunoblotting; IP, immunoprecipitation. Full size image Eogt is required for Dp-dependent cell–matrix interactions Dp is thought to function in maintaining mechanical tension between the apical surface of epithelial cells and the overlying cuticles [22] . As described above, loss of Dp causes defects in the association of the apical surface of the epidermis with the body wall cuticle. However, in other tissues, Dp is not necessary for adhesion of epithelium to the cuticle. In adult wings, inactivation of dp does not affect adhesion between the apical cell surface and the aECM, but instead leads to loss of contact between the basal surfaces of dorsal and ventral epithelium [19] . Furthermore, dp mutation causes overgrowth of the trachea and invagination of the thoracic cuticle at the muscle-attachment sites on the notum (known as vortex and comma phenotypes) possibly because of reduced mechanical tension [22] . However, the molecular mechanisms by which Dp mediates epithelial cell–matrix interactions have not previously been investigated. To assess the functional relevance of biochemical data, the genetic interaction between Eogt and dp was analyzed in the wing. Notably, a single copy of the dp allele markedly increased the penetrance of wing blisters caused by Eogt RNAi in the posterior wing compartment ( Fig. 6a ). Similarly, Eogt and dp interacted to produce vortex and comma phenotypes on the notum ( Fig. 6b ) [23] . Collectively, these data suggest that Eogt is involved in Dp-dependent cell–matrix interactions. 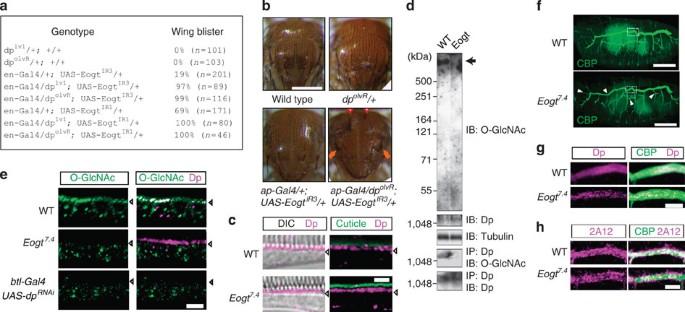Figure 6: EOGT is involved in Dumpy-dependent cell–matrix interactions. (a) Frequency of wing blisters counted in animals of indicated genotype. (b) Genetic interaction betweendpandEogtin vortex (arrow) and comma (arrowhead) phenotypes. These phenotypes were observed only inap-Gal4/dpovlR; UAS-EogtIR3animals. Scale bar, 500 μm. (c) Immunohistochemical analysis for Dp in second-instar tracheae of indicated genotypes. Cuticle autofluorescence is shown in green. Arrowheads mark apical membranes. DIC, differential interference contrast image. Scale bar, 3 μm. (d) Immunoblot analysis of tracheal lysates and the anti-Dp immunoprecipitants prepared from wild-type (WT) andEogt7.4larvae. (e) Immunohistochemical analysis for Dp and O-GlcNAc in second-instar tracheae of indicated genotypes. Arrowheads mark apical membranes. Scale bar, 3 μm. (f) Stage-16 WT andEogtM/Zmutant embryos stained with a fluorescent chitin-binding probe (CBP). Note that tracheal tubes ofEogtM/Zmutant are slightly bent or twisted (arrowheads). Scale bars, 100 μm. (g) Close-ups of dorsal trunk (corresponding to the boxed region in (f)) of stage-15 WT andEogtM/Zembryos stained with anti-Dp antibody (magenta) and chitin-binding probe (green). Scale bar, 10 μm. (h) Stage-15 WT andEogtM/Zembryos were stained with 2A12 (magenta) and chitin-binding probe (green). Data are presented as described in (g). Scale bar, 10 μm. IB, immunoblotting; IP, immunoprecipitation. Figure 6: EOGT is involved in Dumpy-dependent cell–matrix interactions. ( a ) Frequency of wing blisters counted in animals of indicated genotype. ( b ) Genetic interaction between dp and Eogt in vortex (arrow) and comma (arrowhead) phenotypes. These phenotypes were observed only in ap-Gal4/dp ovlR ; UAS-Eogt IR3 animals. Scale bar, 500 μm. ( c ) Immunohistochemical analysis for Dp in second-instar tracheae of indicated genotypes. Cuticle autofluorescence is shown in green. Arrowheads mark apical membranes. DIC, differential interference contrast image. Scale bar, 3 μm. ( d ) Immunoblot analysis of tracheal lysates and the anti-Dp immunoprecipitants prepared from wild-type (WT) and Eogt 7.4 larvae. ( e ) Immunohistochemical analysis for Dp and O-GlcNAc in second-instar tracheae of indicated genotypes. Arrowheads mark apical membranes. Scale bar, 3 μm. ( f ) Stage-16 WT and Eogt M/Z mutant embryos stained with a fluorescent chitin-binding probe (CBP). Note that tracheal tubes of Eogt M/Z mutant are slightly bent or twisted (arrowheads). Scale bars, 100 μm. ( g ) Close-ups of dorsal trunk (corresponding to the boxed region in ( f )) of stage-15 WT and Eogt M/Z embryos stained with anti-Dp antibody (magenta) and chitin-binding probe (green). Scale bar, 10 μm. ( h ) Stage-15 WT and Eogt M/Z embryos were stained with 2A12 (magenta) and chitin-binding probe (green). Data are presented as described in ( g ). Scale bar, 10 μm. IB, immunoblotting; IP, immunoprecipitation. Full size image To address the effect of O-GlcNAcylation on Dp localization and expression, we analyzed larval tracheae while taking advantage of the relative convenience of isolation of mutant tissues for immunohistochemical and biochemical analyses. In wild-type larval tracheae, the apical localization of Dp overlaps or is closely apposed to the cuticles. In contrast, the cuticle co-localization is markedly compromised in the Eogt mutants ( Fig. 6c ). Immunoblot analysis of total lysates prepared from larval tracheae showed that O-GlcNAcylation of Dp is specifically affected in Eogt mutants, while the amount of Dp is not detectably altered ( Fig. 6d ). Accordingly, O-GlcNAc staining of wild-type tracheae detects intracellular O-GlcNAc as well as the apical expression of O-GlcNAc, and the latter is selectively compromised in Eogt mutant cells ( Fig. 6e ). Furthermore, RNAi-induced downregulation of dp resulted in a marked decrease in the apical O-GlcNAc staining ( Fig. 6e ). This suggests that Dp is the major O-GlcNAcylated protein in the tracheal cuticles. Taken together, these results suggest that O-GlcNAcylation is required for the correct localization of Dp in the cuticles, but not for apical secretion in larval tracheae. To further investigate the roles of O-GlcNAcylation for Dp function, we analyzed the embryonic tracheal system in which aECM has an essential role during tracheal tube morphogenesis. In addition to its expected roles in the chitinous matrix, Dp also mediates the cell intercalation that produces unicellular tracheal branches by a mechanism that does not depend on the luminal chitin function [24] , [25] , [26] , [27] . To determine whether O-GlcNAc is required for Dp function during tracheal branching, the tracheal lumen was visualized with a fluorescent probe that labels chitin secreted into the luminal spaces. Analysis of Eogt M/Z embryos with the chitin-binding probe failed to detect the characteristic branch breaks seen in pio or dp mutants ( Fig. 6f ). This lack of requirement for Eogt in chitin-independent activity of Dp is consistent with the idea that O -GlcNAc is required to modulate Dp function associated with chitin in the aECM. Although tracheal networks in Eogt M/Z mutants appear largely intact, the tracheal tubes are slightly twisted or bended and dorsal trunks are occasionally broken ( Fig. 6f ). Since minor defects in tracheal tube morphology were also reported in dp mutants [19] , we investigated the role of O-GlcNAc in Dp distribution in the tracheal lumen. In Eogt mutants, Dp staining revealed an inhomogeneous pattern in comparison to wild-type tracheal tubes, in which Dp staining is largely merged with that of luminal chitins ( Fig. 6g ). In contrast, the staining of 2A12, an uncharacterized luminal antigen, was not altered in the Eogt mutant ( Fig. 6h ), confirming that EOGT does not affect the secretion and distribution of unrelated aECM proteins. These results suggest that O-GlcNAc is required for correct targeting of Dp into the chitinous matrix, possibly by mediating interactions with other components of the aECM. The precise mechanism by which O-GlcNAc mediates cell–matrix interactions must await the elucidation of molecular function of Dp in the aECM. This study demonstrated that O-GlcNAcylation of protein extracellular domains is catalyzed by a novel O-GlcNAc transferase, EOGT, which localizes in the ER. O-GlcNAcylation is a pivotal intracellular modification that regulates a wide range of cellular functions [2] , [6] . Recently, O-GlcNAc was detected on EGF-like repeats of Notch in cultured cells [9] , [28] , although the occurrence and biological function of O-GlcNAcylation in vivo were unknown. We have demonstrated, for the first time, that O-GlcNAc is expressed and functions in the extracellular matrix in animals. Genetic and biochemical analyses revealed that Eogt affects Dp function in wings, notum and larval tracheae. It was also revealed that EOGT-catalyzed O-GlcNAcylation occurs selectively on Dp in total lysates prepared from second-instar larvae. These results suggest that O-GlcNAcylation of Dp is the causative factor accounting for the defective cell–matrix interaction in Eogt phenotypes. However, components of aECM proteins could be altered during developmental stages and distinct molecular mechanisms might underlie the epithelial cell–matrix interaction in the cuticles of different tissues. Thus, we cannot officially exclude the possibility that, under certain circumstances, O-GlcNAcylation occurs on other aECM proteins that would render additional effects on Dp-dependent cell–matrix interactions. Nonetheless, O-GlcNAcylation of Dp is specifically affected in the larval tracheae mutant for Eogt . We therefore propose that EOGT affects cell–matrix interactions by glycosylation of Dp at least in the larval tracheae. O-GlcNAcylation of EGF domains was initially detected on the 20th EGF domain of Notch, which is simultaneously modified with other EGF domain-specific modifications, namely O-fucose and O-glucose. Similar to Notch, Dp also contains a few putative O-fucose and O-glucose modification sites in addition to a large number of potential O-GlcNAcylation sites ( Supplementary Fig. S7 ). Nonetheless, unlike Eogt mutation, genetic inactivation of Ofut1 or rumi (responsible for O-fucosylation and O-glucosylation) did not produce the wing blistering phenotype [13] , [29] , [30] . Thus, O-fucosylation and O-glucosylation, if they occur on Dp, would not be essential for Dp-dependent cell adhesion. On the other hand, Notch signalling is impaired in Ofut1 or rumi mutant by affecting the trafficking, processing and ligand-binding ability of Notch receptors [13] , [30] , [31] , [32] , [33] . In contrast, our study revealed that O-GlcNAc is dispensable for most Notch receptor functions as Eogt mutants do not exhibit any apparent defects in major Notch-dependent processes, such as embryonic neurogenesis, wing margin formation and wing vein specification. Thus, O-GlcNAcylation and O-fucosylation/O-glucosylation are important for distinct protein functions and developmental processes in Drosophila . Nonetheless, there remains the possibility that these O-glycosylations may have partially redundant roles in Dp and Notch function; these may be revealed by simultaneous inactivation of Eogt with rumi or Ofut1 . In summary, our data revealed a novel biochemical mechanism for O-GlcNAcylation of extracellular protein domains in the secretion pathway and the biological function in cell–matrix interactions in Drosophila . Given that Eogt genes are evolutionarily conserved and O-GlcNAcylation motifs are also conserved in several EGF-like domain-containing proteins in mammals, our findings suggest that aberrant cell–matrix or cell–cell interactions caused by dysregulated O-GlcNAcylation may contribute to the aetiology of certain diseases related to the hexosamine signalling pathway. Materials PUGNAc was obtained from Sigma. Drosophila expression vectors encoding EGF20 (pMTBip-EGF20:V5His), Notch EGF repeat-FLAG fusion proteins (pRmHa-N-EGF:FLAG containing 36 EGF-like repeats), GFP tagged with KDEL sequence (pMT-GFP:KDEL) and yeast expression vector encoding EGF20 (pKLAC1-EGF20:V5His) were generated in our previous studies [9] , [14] , [34] . EGF20 C-terminus , C-terminal subdomain of EGF20 was obtained from Biogate. EGF20 C7A,C18A lacking a single disulphide bond of EGF20 was from GenScript. The following antibodies were used: mouse anti-Notch intracellular domain (C17.9C6; dilution 1:1,000; DSHB), mouse anti-V5 (dilution 1:5,000; Invitrogen), mouse anti-α-tubulin (DM1A; dilution 1:5,000; Sigma), mouse anti-FLAG (M2; dilution 1:1,000; Sigma), mouse RL2 (dilution 1:1,000; Abcam), mouse 2A12 (dilution 1:200; DSHB), rat anti-tropomyosin (MAC141; dilution 1:100; Barbraham Institute) and mouse anti-O-GlcNAc (CTD110.6; dilution 1:1,000; Abcam). Polyclonal antibodies raised in rabbit against the peptide CFPRRASENPSKTQRNEL (504–520 amino acids of EOGT) or the peptide CPWQEEPEQPKSNEN (10,755–10,768 amino acids of Dp) were obtained from MBL or GenScript, and used in a 1:500 or 1:1,000 dilution, respectively. Plasmid constructs The plasmids containing Eogt complementary DNA were obtained from the Drosophila Genomics Resource Center (DGRC; Indiana University) and the coding region (nucleotides 189–1,754) was amplified by PCR and cloned into the Bgl II and Xho I sites of pRmHa expression vector (pRmHa-Eogt). The pRmHA-Eogt:V5His vector was constructed, so that the sequence-encoding V5His (LESRGPFEGKPIPNPLLGLDSTRTGHHHHHH) follows after the C-terminus of EOGT. CG9109 and CG31915 were also obtained from DGRC and cloned into pRmHa vector as described above. Using pRmHa-Eogt as a template, FLAG sequence (DYKDDDDK) was introduced by PCR following the instructions of the KOD-Plus-Mutagenesis Kit (Toyobo). The FLAG-tag was inserted after Asp18 (pRmHA-FLAG Asp18 -Eogt) or Asp23 (pRmHA-FLAG Asp23 -Eogt), so that the FLAG-tag still remained on Eogt after cleavage of the signal peptide. Both constructs behave similarly in terms of enzyme activity as well as subcellular localization. Hence, we only showed the results of pRmHA-FLAG Asp18 -Eogt as a representative. FLAG-Eogt ΔRNEL that lacks C-terminal RNEL sequence was generated by PCR as described above using pRmHa-FLAG-Eogt as a template. For constructing expression vectors for Dp, the cDNA fragment corresponding to amino acids 9,377–9,893, 9,908–10,433 or 10,66–11,184 of Dp was amplified by PCR and cloned into the Bgl II/ Xho I sites of pMTBip-V5His vector. These vectors were constructed so that the sequence-encoding V5-His follows after the last amino acid of each protein. For construction of yeast expression vector encoding EGF20 mutants (pKLAC1-EGF20 ΔGlcΔFuc and pKLAC1-EGF20 T34A ), in vitro mutagenesis was performed to mutate the Ser9/Thr17 or Thr34 to Ala. For the Drosophila pUAST-Eogt construct, the Bgl II/ Xho I fragment of Eogt prepared from pRmHa-Eogt was cloned into those sites of pUAST. Three transgenic lines were isolated after injection into Drosophila . They were assayed with tub-Gal4 drivers at 21 °C and exhibited similar phenotypes. Lectin blotting Dp fragments isolated with agarose beads conjugated with anti-V5 antibody (Sigma) were separated by SDS–PAGE, electroblotted to a polyvinylidene difluoride membrane and blocked with Tris buffered saline plus Tween-20 (TBST)-bovine serum albumin (BSA) (10 mM Tris–HCl, pH 7.5, 150 mM NaCl, 0.05% Tween-20 containing 5% BSA). The membrane was incubated overnight at 4 °C with 0.5 mg ml −1 biotinylated succinylated wheat germ agglutinin (Vector) diluted in TBST-BSA. After washing four times with TBST-containing 1 M NaCl, the membrane was incubated for 30 min at room temperature with an avidin-HRP conjugate diluted in TBST-BSA. After washing four times with TBST, the bound lectin was visualized using a chemiluminescent substrate. Transfection and cell staining S2 cells were cultured in Sf-900 II medium (Invitrogen) supplemented with 5% fetal bovine serum. Transient transfection was performed using Cellfectin II (Invitrogen). Protein expression was under the control of an inducible metallothionein promoter and was induced in Sf-900 II supplemented with 0.7 mM CuSO 4 . S2 cells were untreated or treated with PUGNAc (330 μM) for 3 days, followed by transfection with a construct expressing N-EGF:FLAG. The culture media were purified with anti-FLAG M2 beads and detected by immunoblotting. Kc cells were cultured in Schneider's medium (Invitrogen), and the culture media were supplemented or not with 78 mM GlcNAc or glucose and cultured for 24 h ( Fig. 3a ). Total cell lysates or the immunoprecipitants were separated by SDS–PAGE, transferred to Immobilon-P transfer membranes (Millipore), probed with CTD110.6 to detect O-GlcNAc or appropriate primary antibodies, and visualized using HRP-labeled secondary antibodies and a chemiluminescent substrate. Tissue culture slides (eight chamber; Nunc) were coated for at least 2 h with 0.5 mg ml −1 of Concanavalin A (from Canavalia ensiformis ; Sigma). S2 cells were plated on Concanavalin A-treated slides and allowed to spread out on the slide for 1–2 h (ref. 35 ). Cells were fixed for 10 min with 4% formaldehyde (Polysciences Inc.), permeabilized with PBST-BSA (PBS containing 0.1% Triton X-100 and 1% BSA), and incubated with appropriate antibodies in PBST-BSA. dsRNA preparation and RNAi RNAi for S2 cells were performed by adding dsRNA to Sf-900 II serum-free medium followed by culturing in Sf-900 II medium supplemented with 2.5% fetal bovine serum for additional 4 days as described previously [9] , [36] . For the production of dsRNA for Eogt , transcription templates (nucleotides 197–1,044) were generated by PCR such that they contained T7 promoters on each end of the template. The primer sets used for PCR are as follows: T7-Eogt-Fw 5′- TAATACGACTCACTATAGGG GCCAATCCTGCCAATACTC-3′; T7-Eogt-Rv : 5′- TAATACGACTCACTATAGGG GCGAGAAGGCCTTAAATGTG-3′, where the T7 sequence is underlined. Purified PCR products were used as the templates for in vitro transcription reactions using a Megascript RNAi kit (Ambion). Drosophila stocks BG00673 was obtained from Bloomington stock center. Eogt LL00272 FRT40A , dp olvR and dp lv1 were obtained from the DGRC. Gal4 drivers used were ap-Gal4 (Flybase ID; Fbti0009983), tub-Gal4 (DGRC) and en-Gal4 (A. Brand). Eogt LL00272 contains a modified piggyBac transposon with splice traps [37] within the 5′-UTR, located 87 bp upstream of the Eogt translation start site. Drosophila RNAi lines UAS-Eogt IR1 (9867R-1) UAS-Eogt IR3 (9867R-3), and UAS-dp IR (15637R-1) were obtained from the National Institute of Genetics (Mishima, Japan). Drosophila crosses For generation of clones of cells mutant for Eogt in the wing disc, Eogt 7.4 was crossed with FRT40A by meiotic recombination, and mutant clones were generated by crossing to y w hs-flp 122 ; ubi-GFP:nls FRT40A flies and heat shocking to induce flippase-mediated mitotic recombination [38] . For generation of marked clones in the adult wing disc, Eogt 7.4 ck FRT40A/CyO was used for flippase-mediated mitotic recombination. To obtain mutants lacking both maternal and zygotic Eogt (Eogt M/Z ), germline clones of Eogt 7.4 were made by crossing hs-flp; Eogt 7.4 FRT40A / CyO virgins to ovoD FRT40A / CyO males and heat shocking the progeny at 38 °C for 1 h on two successive days during the first and second larval instar. Then, hs-flp ; Eogt 7.4 FRT40A / ovoD FRT40A female progeny that contained Eogt 7.4 germline clones were crossed to Eogt 7.4 /CyO; twi-Gal4 UAS-GFP males. All animals were raised at 25 °C unless otherwise specified. Mutation of Eogt BG00673 contains an insertion of a P transposable element within the 5′-UTR, located 160 bp upstream of the Eogt translation start site. This P-element insertion line is homozygous-viable and fertile, and shows no visible phenotype. The deletions of genomic DNA of Eogt 7.4 and Eogt 34.2 were generated by imprecise excision of BG00673 . All the mutated alleles result in larval lethality in different allelic combinations. The lethality associated with homozygous Eogt 7.4 mutations can be rescued by ubiquitous expression of UAS - Eogt under the control of the tub-Gal4 driver. RNAi in Drosophila The RNAi phenotypes of Eogt were rescued by mouse EOGT expression, excluding the possibility of off-target effects of RNAi. btl-Gal4 / UAS-dp IR larvae were raised at 28 °C. All other progeny were raised at 25 °C unless otherwise specified. Tissue staining Embryos and larval tissues were fixed in 4% paraformaldehyde and stained with antibodies as described previously [29] . For phalloidin staining, embryos were devitellenized in 80% ethanol instead of methanol. In situ hybridization in whole-mount Drosophila embryos was carried out using in vitro -transcribed Eogt (nucleotides 197–1,044) [29] . Chitin staining was performed using FITC-conjugated chitin-binding probe (New England Biolabs). Preparation of larval extracts for immunoprecipitation of Dp Wild-type or Eogt 7.4 early second-instar larvae were washed twice with PBS, and then homogenized in PBS. After extraction with a high-salt buffer (8.5% NaCl) containing 1% dodecyl-maltoside, the insoluble materials containing larval cuticles were dissolved in lysis buffer (1% Nonidet P-40, 0.06% SDS, 20 mM HEPES, pH 7.5). The lysates were immunoprecipitated at 4 °C for 2 h using Protein G Sepharose (GE Healthcare) and the anti-Dp antibody as described above. Transmission electron microscopy The second-instar larvae were dissected between the A6 and A7 segments, fixed with 4% paraformaldehyde and 1% glutaraldehyde in cacodylate buffer (pH 7.4) [39] , and observed by transmission electron microscopy [40] . Enzyme activity assay Membrane fraction proteins were prepared as described [34] and further purified with Ni-magnetic beads (Promega). O-GlcNAc transferase assay was performed in the glycosylation buffer (200 mM HEPES-NaOH, pH 7.0, 1 mM MnCl 2 , 1 mg ml −1 BSA) containing 2 μM UDP-[ 3 H]GlcNAc (60 Ci mmol −1 ; ARC), 1 μg of EGF20-V5His and affinity-purified EOGT as an enzyme source in a volume of 20 μl. After incubation at 25 °C for 30 min, the reaction sample was applied to a LC-18 SPE tube (Supelco), washed and eluted with 1 ml of 80% acetonitrile, 0.052% trifluoroacetic acid. Radioactivity was measured by liquid scintillation counting. Accession codes: The nucleotide sequence has been submitted to the DNA databank of Japan with accession number AB675601 . How to cite this article: Sakaidani, Y. et al . O-Linked- N -acetylglucosamine on extracellular protein domains mediates epithelial cell–matrix interactions. Nat. Commun. 2:583 doi: 10.1038/ncomms1591 (2011).